Effector lymphocyte-induced lymph node-like vasculature enables naive T-cell entry into tumours and enhanced anti-tumour immunity The presence of lymph node (LN)-like vasculature in tumours, characterized by expression of peripheral node addressin and chemokine CCL21, is correlated with T-cell infiltration and positive prognosis in breast cancer and melanoma patients. However, mechanisms controlling the development of LN-like vasculature and how it might contribute to a beneficial outcome for cancer patients are unknown. Here we demonstrate that LN-like vasculature is present in murine models of melanoma and lung carcinoma. It enables infiltration by naive T cells that significantly delay tumour outgrowth after intratumoral activation. Development of this vasculature is controlled by a mechanism involving effector CD8 T cells and NK cells that secrete LTα 3 and IFNγ. LN-like vasculature is also associated with organized aggregates of B lymphocytes and gp38 + fibroblasts, which resemble tertiary lymphoid organs that develop in models of chronic inflammation. These results establish LN-like vasculature as both a consequence of and key contributor to anti-tumour immunity. Lymph nodes (LNs) contain specialized blood vessels called high endothelial venules (HEVs). HEVs display peripheral node addressin (PNAd) and CCL21, and mediate entry of naive and memory T cells expressing the cognate ligands L-selectin and CCR7 (ref. 1 ). HEVs are not normally found outside lymphoid tissue but are induced at sites of chronic inflammation [2] . They have been recently detected in human tumours and are associated with a positive prognosis [3] , [4] , [5] , [6] . This suggests that PNAd and CCL21 on tumour vasculature are important elements of immunological tumour control, but the mechanisms inducing their expression and their function in supporting anti-tumour immunity are unknown. In peripheral LN, HEV morphology and adhesion molecule expression are maintained by dendritic cells (DCs) that express lymphotoxin (LT) α 1 β 2 , which acts via the LTβ receptor (LTβR) on blood endothelial cells [7] , [8] . In inflamed non-lymphoid tissues, PNAd and CCL21 expression is often associated with the development of organized structures resembling LN termed tertiary lymphoid organs (TLOs). Control of PNAd in TLOs is thought to be similar to control in LN. Inhibiting LTβR signalling blocks PNAd expression in many TLO models [9] , [10] , [11] , [12] and DCs regulate the presence of PNAd + vasculature and associated TLO in inflamed lungs [13] , [14] . PNAd + vasculature can be induced by transgenic expression of LTα and LTβ in the pancreas and kidney [15] , [16] , or by transgenic expression of CCL21 in the pancreas and thyroid via an LTβR-dependent pathway [17] , [18] . Similarly, transgenic expression of LTα or CCL21 in tumours leads to induction of PNAd + vasculature [19] , [20] , [21] . However, these transgenic models do not allow one to determine the mechanisms regulating spontaneously arising PNAd + vasculature. In non-transgenic tumour models, the density of intratumoral DCs [22] and regulatory T-cell (Treg) depletion [23] have been associated with the presence of LN-like vasculature, but the mechanisms controlling its development remain unknown. Although it is generally assumed that tumour-infiltrating CD8 T cells are effector cells that differentiated in tumour-draining LN, we previously showed that naive T cells also infiltrate tumours [24] . Tumour-infiltrating naive T cells differentiate into functional effector cells in the tumour [24] and promote its destruction [25] , [26] . However, this work did not establish the mechanisms that supported naive T-cell entry. Here we investigated this using murine tumour models established in the absence of transgenic expression of chemokines or cytokines. We show that tumours spontaneously develop LN-like vasculature and identify novel molecular mechanisms, dependent on endogenous effector lymphocytes that drive its formation. We also demonstrate that LN-like vasculature is the major portal through which naive T cells enter tumours, and that infiltrating naive T cells are able to delay tumour outgrowth. These findings place intratumoral LN-like vasculature in a positive feedback loop that is both a consequence of and contributor to anti-tumour immunity. Tumours develop LN-like vasculature Recent studies have identified LN-like vasculature in human tumours as a prognostic marker of enhanced patient survival [3] , [4] , [5] , [6] . Thus, we evaluated whether similar vessels developed in murine tumours. By immunofluorescence, we detected PNAd on CD31 + endothelium in subcutaneous (s.c.) and intraperitoneal (i.p.) B16-OVA tumours in C57BL/6 mice ( Fig. 1a–c ; low-power images in Supplementary Fig. 1a,b ). No staining was observed with isotype control antibody ( Fig. 1c ). PNAd was also expressed on vasculature of OVA-expressing Lewis lung carcinoma tumours (LLC-OVA) and B16 expressing a tyrosinase epitope as a model antigen (B16-AAD), in both s.c. and i.p. locations ( Fig. 1d–g ). The fraction of PNAd + vessels in tumours ( ∼ 5–10%) was much smaller than in LN ( Fig. 1h ). PNAd detection on tumour vasculature also required tyramide amplification, while detection on LN HEV did not, indicating a significantly lower level of expression. In i.p. tumours, a fraction of PNAd + endothelial cells exhibited the cuboidal morphology typical of LN HEV, with PNAd apparent at both the luminal and abluminal surfaces ( Fig. 1i,j ). Otherwise, PNAd was expressed on endothelial cells with a flat morphology, typical of the overall tumour vasculature ( Fig. 1a,b ). To verify that PNAd was expressed on the luminal surface, we injected MECA-79 antibody intravenously (i.v.) before tumour harvest. This labelled the majority of LN HEVs and tumour vessels, which in serial sections were PNAd + , based on our standard staining protocol ( Fig. 1k,l ). No luminal staining was detected after injecting an isotype control antibody (unpublished). In both tumour sites, PNAd + vessels coexpressed MAdCAM-1 and VCAM-1 ( Supplementary Fig. 1c–g ). However, VCAM-1 was expressed more highly on PNAd-negative vessels. In i.p. but not in s.c. tumours, there were also many vessels that expressed MAdCAM-1 without PNAd ( Supplementary Fig. 1e–g ). PNAd + vasculature was also present in genetically induced melanomas from BRAF V600E PTEN −/− transgenic mice [27] ( Supplementary Fig. 2a ). 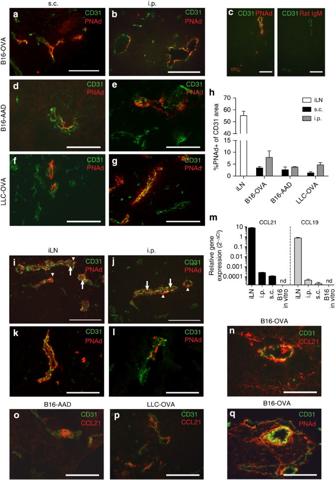Figure 1: Tumours spontaneously develop LN-like vasculature expressing PNAd and CCL21. Frozen sections of day 14 B16-OVA tumours (a–c), B16-AAD tumours (d,e) or LLC-OVA tumours (f,g) growing s.c. (a,d,f) and i.p. (b,c,e,g) in C57BL/6 mice were stained for CD31 and PNAd. Inc, two adjacent sections were stained for CD31 and with either PNAd or Rat IgM isotype control antibody. (h) The percentage of CD31+area expressing PNAd in each tissue was quantified as described in Methods. iLN, inguinal LN. Bars represent mean+s.e.m.n=4 per tissue. PNAd staining on HEV in iLN (i,k) and i.p. B16-OVA tumours (j,l). Ini,j, arrows mark luminal PNAd, arrowheads mark abluminal PNAd. Ink,l, luminal PNAd was detected with streptavidin after i.v. injection of biotinylated MECA-79 antibody 30 min before harvest. (m) Expression ofCcl21,Ccl19andHprtmRNA inin vitroB16-cOVA cultures, and lysates (n=3) of s.c. and i.p. B16-cOVA tumours and iLN was detected using 40-cycle reverse transcriptase–PCR. Relative gene expression is presented as 2^-ΔCTrelative to HPRT. (n–q) Sections of i.p. B16-OVA tumours (n,q), B16-AAD tumours (o) or LLC-OVA tumours (p) were stained for CD31, and either CCL21 (n–p) or PNAd (q). Two adjacent sections are shown innandq. All images are representative of at least three independent experiments. Scale bars=100 μm. Figure 1: Tumours spontaneously develop LN-like vasculature expressing PNAd and CCL21. Frozen sections of day 14 B16-OVA tumours ( a – c ), B16-AAD tumours ( d , e ) or LLC-OVA tumours ( f , g ) growing s.c. ( a , d , f ) and i.p. ( b , c , e , g ) in C57BL/6 mice were stained for CD31 and PNAd. In c , two adjacent sections were stained for CD31 and with either PNAd or Rat IgM isotype control antibody. ( h ) The percentage of CD31 + area expressing PNAd in each tissue was quantified as described in Methods. iLN, inguinal LN. Bars represent mean+s.e.m. n =4 per tissue. PNAd staining on HEV in iLN ( i , k ) and i.p. B16-OVA tumours ( j , l ). In i , j , arrows mark luminal PNAd, arrowheads mark abluminal PNAd. In k , l , luminal PNAd was detected with streptavidin after i.v. injection of biotinylated MECA-79 antibody 30 min before harvest. ( m ) Expression of Ccl21 , Ccl19 and Hprt mRNA in in vitro B16-cOVA cultures, and lysates ( n =3) of s.c. and i.p. B16-cOVA tumours and iLN was detected using 40-cycle reverse transcriptase–PCR. Relative gene expression is presented as 2^-ΔC T relative to HPRT. ( n – q ) Sections of i.p. B16-OVA tumours ( n , q ), B16-AAD tumours ( o ) or LLC-OVA tumours ( p ) were stained for CD31, and either CCL21 ( n – p ) or PNAd ( q ). Two adjacent sections are shown in n and q . All images are representative of at least three independent experiments. Scale bars=100 μm. Full size image We also detected messenger RNA for chemokines Ccl21 and Ccl19 in s.c. and i.p. tumour lysates, although at lower levels than in LN ( Fig. 1m ). B16-OVA cells cultured in vitro did not express detectable levels of either chemokine. CCL21 protein was displayed on the vasculature of all tumours evaluated ( Fig. 1n–p ), but CCL19 protein was undetectable, probably reflecting the ∼ 10-fold lower expression levels ( Fig. 1m ). Staining serial sections established that CCL21 was coexpressed on PNAd + vessels ( Fig. 1q ). Thus, multiple murine tumour models spontaneously develop LN-like vasculature expressing PNAd and CCL21. LN-like vasculature enables naive T-cell infiltration We previously showed that naive T cells directly infiltrated tumours [24] ; thus, we tested whether LN-like vasculature served as their entry point. We transferred naive Thy1.1 congenic OT-I cells into C57BL/6 mice with established s.c. or i.p. B16-OVA tumours and evaluated the absolute number of infiltrating OT-I cells after 1 or 18 h. This number was consistent across experiments and largely independent of tumour size (unpublished observations). We used 18 h as a standard time point for most of our experiments, in keeping with other studies [28] , [29] , [30] , [31] . However, infiltration was largely complete by 1 h ( Fig. 2a ). Co-transferred naive (CD44 lo ) polyclonal T cells infiltrated tumours equivalently to naive OT-I cells, demonstrating that infiltration was not dependent on antigen specificity ( Fig. 2b ). The efficiency of naive T-cell infiltration into tumours was lower than that into LN; however, it was consistent with the lower PNAd expression on tumour vasculature ( Fig. 2c ). 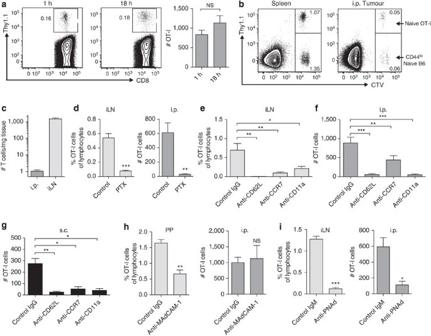Figure 2: LN-like vasculature supports naive T-cell infiltration. (a) Representative plots and summary data (n=3) for naive T-cell infiltration. Naive Thy1.1+OT-I cells (4 × 106) were injected i.v. into WT mice with established i.p. B16-OVA tumours. One or 18 h after transfer, tumours were harvested and infiltrating naive T cells were enumerated by flow cytometry. Numbers indicate the percentage of naive OT-I cells out of the live singlet CD45+CD8+parent gate. (b) WT mice with i.p. B16-OVA tumours received a 50:50 mix of Cell Trace Violet (CTV)-labelled naive Thy1.1+OT-I cells and CD44lonaive T cells from C57BL/6 mice i.v. (4 × 106total cells). Infiltration into tissues was determined after 18 h. (c) Homing efficiency (number of T cells per mg tissue) of naive OT-I cells to i.p. tumours and iLN.n=7. Naive OT-I cells pretreated with pertussis toxin (PTX) (d) or antibodies against L-selectin (CD62L), CCR7 or LFA-1 (CD11a) (e–g) were transferred into tumour-bearing mice. Infiltration into iLN (d,e), i.p. (d,f) or s.c. (g) B16-OVA tumours was determined after 18 h.n=10–17 per group (tumours) or 4 per group (iLN). Naive OT-I cells were transferred into WT mice with i.p. B16-OVA tumours pre-treated with anti-MAdCAM-1 antibody or Rat IgG isotype control (h), or anti-PNAd antibody or Rat IgM isotype control (i). Infiltration into tissues was determined 1 h after T-cell transfer.n=5 (h) or 3(i). PP, Peyer’s patches; iLN, inguinal lymph node. Data (mean+s.e.m.) are pooled from two independent experiments. ns:P>0.05, *P<0.05, **P<0.01, ***P<0.001 by unpairedt-test (a,c,h,i) or one-way analysis of variance with Dunnett’s post test (e–g). Figure 2: LN-like vasculature supports naive T-cell infiltration. ( a ) Representative plots and summary data ( n =3) for naive T-cell infiltration. Naive Thy1.1 + OT-I cells (4 × 10 6 ) were injected i.v. into WT mice with established i.p. B16-OVA tumours. One or 18 h after transfer, tumours were harvested and infiltrating naive T cells were enumerated by flow cytometry. Numbers indicate the percentage of naive OT-I cells out of the live singlet CD45 + CD8 + parent gate. ( b ) WT mice with i.p. B16-OVA tumours received a 50:50 mix of Cell Trace Violet (CTV)-labelled naive Thy1.1 + OT-I cells and CD44 lo naive T cells from C57BL/6 mice i.v. (4 × 10 6 total cells). Infiltration into tissues was determined after 18 h. ( c ) Homing efficiency (number of T cells per mg tissue) of naive OT-I cells to i.p. tumours and iLN. n =7. Naive OT-I cells pretreated with pertussis toxin (PTX) ( d ) or antibodies against L-selectin (CD62L), CCR7 or LFA-1 (CD11a) ( e – g ) were transferred into tumour-bearing mice. Infiltration into iLN ( d , e ), i.p. ( d , f ) or s.c. ( g ) B16-OVA tumours was determined after 18 h. n =10–17 per group (tumours) or 4 per group (iLN). Naive OT-I cells were transferred into WT mice with i.p. B16-OVA tumours pre-treated with anti-MAdCAM-1 antibody or Rat IgG isotype control ( h ), or anti-PNAd antibody or Rat IgM isotype control ( i ). Infiltration into tissues was determined 1 h after T-cell transfer. n =5 ( h ) or 3( i ). PP, Peyer’s patches; iLN, inguinal lymph node. Data (mean+s.e.m.) are pooled from two independent experiments. ns: P >0.05, * P <0.05, ** P <0.01, *** P <0.001 by unpaired t -test ( a , c , h , i ) or one-way analysis of variance with Dunnett’s post test ( e – g ). Full size image Disruption of chemokine signalling in transferred naive OT-I cells by pertussis toxin pretreatment prevented their infiltration into tumours ( Fig. 2d ), indicating entry is chemokine dependent. To directly determine whether naive T-cell infiltration required interactions with LN-like vasculature, OT-I cells were pretreated with either anti-L-selectin or anti-CCR7 blocking antibodies before adoptive transfer. T-cell entry into LN and both s.c. and i.p. tumours was significantly inhibited when either molecule was blocked ( Fig. 2e–g ). CCR7 signalling activates integrin LFA-1 to cause arrest and extravasation via interactions with ICAM-1 (ref. 32 ). ICAM-1 was widely expressed on tumour vessels (unpublished observations) and pretreatment of naive OT-I cells with anti-CD11a to block LFA-1 also prevented infiltration into both LN and tumours ( Fig. 2e–g ). To determine whether infiltration was mediated by L-selectin binding to MAdCAM-1 or PNAd, we transferred OT-I cells into i.p. tumour-bearing mice pretreated to block luminally expressed molecules with injection of either anti-MAdCAM-1, anti-PNAd or isotype control. MAdCAM-1 blockade reduced infiltration into Peyer’s patches but had no effect on tumour infiltration ( Fig. 2h ). In contrast, blockade of luminal PNAd abolished naive T-cell infiltration into both inguinal LN and tumours ( Fig. 2i ). These results demonstrate that naive T cells infiltrate tumours by adhering to PNAd + vasculature. PNAd and CCL21 in tumours do not require LTβR signalling Luminal PNAd expression on LN HEVs is primarily controlled by LTβR signalling [8] . To determine whether this pathway controlled PNAd in tumours, we blocked it throughout i.p. tumour outgrowth, using a LTβR-Ig fusion protein [25] . This did not affect overall LN vascularity ( Fig. 3a,b ), but significantly decreased PNAd expression on LN vessels and resulted in loss of HEV morphology ( Fig. 3a,c ). As expected, residual PNAd on flat endothelium in LTβR-blocked mice was abluminal, whereas PNAd on control HEV was displayed on both luminal and abluminal surfaces ( Fig. 3a ). In a parallel group of LTβR-Ig-treated mice that received naive OT-I T-cells, loss of luminal PNAd led to significantly reduced LN infiltration ( Fig. 3d ). However, LTβR-Ig blockade had no effect on PNAd expression on i.p. tumour vasculature ( Fig. 3e–g ). Concordantly, naive OT-I cells transferred to a parallel cohort of LTβR-blocked animals entered i.p. tumours in greater numbers than controls, demonstrating that PNAd was still expressed on the luminal surface ( Fig. 3h ). LTβR-Ig treatment did not alter expression of Ccl21 in either LN or tumours ( Fig. 3i,j ). Thus, the mechanisms that control luminal PNAd on LN HEV and tumour vasculature are distinct. 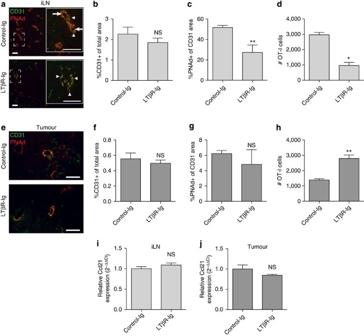Figure 3: Expression of PNAd and CCL21 in B16-OVA tumours does not require LTβR signalling. (a–c) Expression of CD31 and PNAd in inguinal LN from control-Ig or LTβR-Ig-treated mice. (a) Boxed area is shown in inset. Arrows mark luminal PNAd, arrowheads mark abluminal PNAd. Percentages of total area positive for CD31 (b) and of the CD31 area positive for PNAd (c) were calculated as described in Methods.n=4–5 per group (b) or 9–10 per group (c). (d) Infiltration of naive OT-I cells into inguinal LN of control-Ig and LTβR-Ig-treated mice determined as inFig. 2.n=3. (e–g) Expression of CD31 and PNAd in i.p. tumours from control-Ig or LTβR-Ig-treated mice. Expression was analysed in mice that did not receive naive OT-I T cells.n=5 per group. (h) Infiltration of naive OT-I cells into i.p. tumours of control-Ig and LTβR-Ig-treated mice.n=5 per group. Expression ofCcl21in LN (i) and i.p. tumour (j) lysates was determined by quantitative reverse transcriptase–PCR. Results were calculated by the ΔΔCTmethod relative to HPRT with expression levels in control samples normalized to 1.n=≥3 per group. Data (mean+s.e.m.) are representative of two independent experiments. ns:P>0.05, *P<0.05, **P<0.01 by unpairedt-test. Scale bars=100 μm. Figure 3: Expression of PNAd and CCL21 in B16-OVA tumours does not require LTβR signalling. ( a – c ) Expression of CD31 and PNAd in inguinal LN from control-Ig or LTβR-Ig-treated mice. ( a ) Boxed area is shown in inset. Arrows mark luminal PNAd, arrowheads mark abluminal PNAd. Percentages of total area positive for CD31 ( b ) and of the CD31 area positive for PNAd ( c ) were calculated as described in Methods. n =4–5 per group ( b ) or 9–10 per group ( c ). ( d ) Infiltration of naive OT-I cells into inguinal LN of control-Ig and LTβR-Ig-treated mice determined as in Fig. 2 . n =3. ( e – g ) Expression of CD31 and PNAd in i.p. tumours from control-Ig or LTβR-Ig-treated mice. Expression was analysed in mice that did not receive naive OT-I T cells. n =5 per group. ( h ) Infiltration of naive OT-I cells into i.p. tumours of control-Ig and LTβR-Ig-treated mice. n =5 per group. Expression of Ccl21 in LN ( i ) and i.p. tumour ( j ) lysates was determined by quantitative reverse transcriptase–PCR. Results were calculated by the ΔΔC T method relative to HPRT with expression levels in control samples normalized to 1. n =≥3 per group. Data (mean+s.e.m.) are representative of two independent experiments. ns: P >0.05, * P <0.05, ** P <0.01 by unpaired t -test. Scale bars=100 μm. Full size image CD8 T cells induce LN-like vasculature in i.p. tumours To elucidate mechanisms underlying the development of LN-like vasculature in tumours, we investigated whether immune cell subsets were involved. Infiltration of transferred naive OT-I and naive polyclonal T-cells into i.p. tumours growing in Rag2 −/− mice, which lack endogenous B and T lymphocytes, was significantly decreased ( Fig. 4a,b ). However, naive T-cells infiltrated i.p. tumours grown in B-cell-deficient μMT −/− mice normally ( Fig. 4c ). Furthermore, infiltration into i.p. tumours in β2M −/− mice, which retain B cells and CD4 T cells but lack endogenous CD8 T cells and natural killer (NK) T cells, was poor ( Fig. 4b ). However, infiltration into i.p. tumours in CD1d −/− mice was normal, ruling out a requirement for NKT cells and pinpointing CD8 T cells as necessary ( Fig. 4d ). A role for CD8 T cells in induction of LN-like vasculature was also suggested in genetically induced melanomas from BRAF V600E PTEN −/− transgenic mice. These tumours are well infiltrated by endogenous CD8 T cells [33] and the majority contained PNAd + vasculature ( Supplementary Fig. 2b ). In contrast, tumours from BRAF V600E PTEN −/− mice with an activating mutation in β-catenin [34] are devoid of infiltrating CD8 T cells [35] and none of these tumours contained PNAd + vasculature ( Supplementary Fig. 2b ). 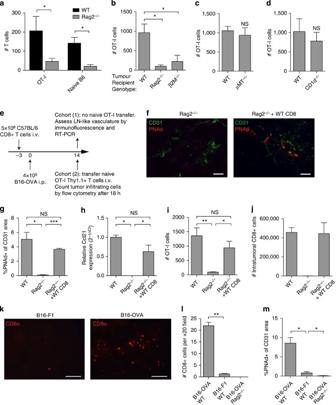Figure 4: Endogenous CD8 T-cells induce LN-like vasculature in i.p. tumours. (a) Infiltration of naive Thy1.1+OT-I cells and CD44lonaive polyclonal T cells purified from C57BL/6 and co-transferred into WT orRag2−/−mice with established i.p. B16-OVA tumours was determined after 18 h by flow cytometry.n=3 per genotype. Infiltration of naive OT-I cells into i.p. B16-OVA tumours in the indicated mice was determined.n=3 (b) or 5 (c,d). (e) Experimental protocol used for the repletion ofRag2−/−mice with CD8 T cells before tumour implantation. On day 14 after tumour implantation, tumours from one cohort of mice were harvested for immunofluorescence and reverse transcriptase–PCR. A second cohort of mice received naive OT-I cells and tumours were processed for flow cytometry to assess infiltration into tumours. Representative images (f) and summary data (g,n=3–4) for PNAd expression in tumours in the indicated mice. (h)Ccl21expression (n=2) in i.p. tumour lysates was quantified as inFig. 3. (i) Infiltration of naive OT-I cells into i.p. B16-OVA tumours in the indicated mice was determined.n=3–5 per group. (j) The absolute number of endogenous (non-OT-I) CD8+T cells that had accumulated in day 14 i.p. B16-OVA tumours in mice with the indicated background was determined by flow cytometry. Representative images (k) and summary data (l,n=2) for endogenous CD8 T-cell accumulation in day 14 B16-F1 or B16-OVA tumours growing in WT mice determined by immunofluorescence. (m) Expression of PNAd in either B16-F1 or B16-OVA tumours growing in the indicated mice.n=4 per group. Data (mean+s.e.m.) are representative of at least two independent experiments. ns:P>0.05, *P<0.05, **P<0.01, ***P<0.001 by unpairedt-test (a,c,d) or one-way analysis of variance with Tukey’s post test (b,g–m). Figure 4: Endogenous CD8 T-cells induce LN-like vasculature in i.p. tumours. ( a ) Infiltration of naive Thy1.1 + OT-I cells and CD44 lo naive polyclonal T cells purified from C57BL/6 and co-transferred into WT or Rag2 −/− mice with established i.p. B16-OVA tumours was determined after 18 h by flow cytometry. n =3 per genotype. Infiltration of naive OT-I cells into i.p. B16-OVA tumours in the indicated mice was determined. n =3 ( b ) or 5 ( c , d ). ( e ) Experimental protocol used for the repletion of Rag2 −/− mice with CD8 T cells before tumour implantation. On day 14 after tumour implantation, tumours from one cohort of mice were harvested for immunofluorescence and reverse transcriptase–PCR. A second cohort of mice received naive OT-I cells and tumours were processed for flow cytometry to assess infiltration into tumours. Representative images ( f ) and summary data ( g , n =3–4) for PNAd expression in tumours in the indicated mice. ( h ) Ccl21 expression ( n =2) in i.p. tumour lysates was quantified as in Fig. 3 . ( i ) Infiltration of naive OT-I cells into i.p. B16-OVA tumours in the indicated mice was determined. n =3–5 per group. ( j ) The absolute number of endogenous (non-OT-I) CD8 + T cells that had accumulated in day 14 i.p. B16-OVA tumours in mice with the indicated background was determined by flow cytometry. Representative images ( k ) and summary data ( l , n =2) for endogenous CD8 T-cell accumulation in day 14 B16-F1 or B16-OVA tumours growing in WT mice determined by immunofluorescence. ( m ) Expression of PNAd in either B16-F1 or B16-OVA tumours growing in the indicated mice. n =4 per group. Data (mean+s.e.m.) are representative of at least two independent experiments. ns: P >0.05, * P <0.05, ** P <0.01, *** P <0.001 by unpaired t -test ( a , c , d ) or one-way analysis of variance with Tukey’s post test ( b , g – m ). Full size image To directly establish the importance of endogenous CD8 T cells, we reconstituted Rag2 −/− mice with total CD8 T cells purified from C57BL/6 mice before implantation of i.p. tumours. We then assessed development of LN-like vasculature directly by measuring expression of PNAd and CCL21, and indirectly by monitoring infiltration of transferred naive OT-I cells, in separate cohorts of mice ( Fig. 4e ). PNAd was completely absent from i.p. tumour vasculature in Rag2 −/− mice and expression of Ccl21 was significantly decreased ( Fig. 4f–h ). In i.p. tumours from CD8-repleted Rag2 −/− mice, however, expression of PNAd and Ccl21 , and infiltration of transferred naive OT-I cells were restored to levels seen in wild-type (WT) mice ( Fig. 4f–i ). It seemed likely to be that this was directly mediated by CD8 effector T cells from the repleting pool that had infiltrated the tumour, because equivalent numbers of endogenous CD8 T cells were found in tumours in repleted Rag2 −/− mice and C57BL/6 mice ( Fig. 4j ). In keeping with this, B16-F1 tumours, which lack a strong antigen, show reduced infiltration by endogenous CD8 T cells in C57BL/6 mice, compared with B16-OVA tumours ( Fig. 4k,l ). In addition, PNAd expression on B16-F1 tumour vasculature was significantly lower than on B16-OVA vasculature, but still greater than in B16-OVA tumours from Rag2 −/− mice ( Fig. 4m ). These data establish that PNAd and CCL21 expression on i.p. tumour vasculature is determined by the extent of infiltration of endogenous effector CD8 T cells, which is in turn related to the strength of the antigenic stimulus that activates them. T and NK cells induce LN-like vasculature in s.c. tumours In contrast to i.p. tumours, transferred naive OT-I cells infiltrated s.c. tumours in control and Rag2 −/− mice equivalently, whereas s.c. tumours in β2M −/− hosts continued to be poorly infiltrated ( Fig. 5a ). This suggested that NK cells, which are hyporesponsive in β2M −/− but not Rag2 −/− animals [36] , [37] , acted redundantly with endogenous CD8 T cells to induce LN-like vasculature in s.c. tumours. Indeed, although depletion of NK cells from WT mice had no effect, naive T-cell infiltration into s.c. tumours was significantly diminished when NK cells were depleted from Rag2 −/− mice and restored in NK-depleted Rag2 −/ − mice reconstituted with CD8 T cells ( Fig. 5b,c ). In addition, PNAd and Ccl21 expression was significantly decreased in s.c. tumours from NK-depleted Rag2 −/− mice ( Fig. 5d–f ). Therefore, NK cells act redundantly with endogenous CD8 T cells to induce LN-like vasculature in s.c. tumours. 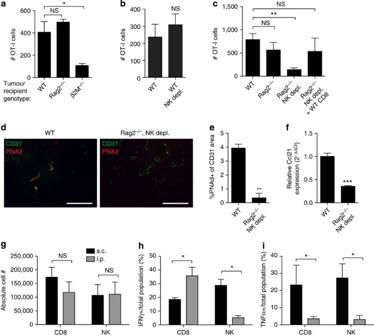Figure 5: CD8 T cells and NK cells act redundantly to induce LN-like vasculature in s.c. tumours. (a–c) Infiltration of naive OT-I cells into s.c. B16-OVA tumours in the indicated mice was determined as inFig. 2.n=3 (a) or 5–8 (b,c) per group. Representative images (d) and summary data (e,n=3) for PNAd expression in tumours in the indicated mice. (f)Ccl21expression (n=3) in s.c. tumour lysates was quantified as inFig. 3. (g) Number of endogenous CD8 T cells (CD3+CD8+) and NK cells (CD3−CD4−NK1.1+) present in s.c. (black bars) and i.p. (grey bars) tumours in WT mice was determined by flow cytometry.n≥8 per group. The percentage of total CD8 T cells or NK cells producing IFNγ (h) or TNFα (i) in s.c. (black bars) or i.p. (grey bars) tumours from WT mice was assessed by intracellular staining 4 h after Brefeldin A injection.n=3–5 per group. Data (mean+s.e.m.) are representative of at least two independent experiments. ns:P>0.05, *P<0.05, **P<0.01, ***P<0.001 by unpairedt-test (b,e–i) or one-way analysis of variance with Dunnett’s post test (a,c). Figure 5: CD8 T cells and NK cells act redundantly to induce LN-like vasculature in s.c. tumours. ( a – c ) Infiltration of naive OT-I cells into s.c. B16-OVA tumours in the indicated mice was determined as in Fig. 2 . n =3 ( a ) or 5–8 ( b , c ) per group. Representative images ( d ) and summary data ( e , n =3) for PNAd expression in tumours in the indicated mice. ( f ) Ccl21 expression ( n =3) in s.c. tumour lysates was quantified as in Fig. 3 . ( g ) Number of endogenous CD8 T cells (CD3 + CD8 + ) and NK cells (CD3 − CD4 − NK1.1 + ) present in s.c. (black bars) and i.p. (grey bars) tumours in WT mice was determined by flow cytometry. n ≥8 per group. The percentage of total CD8 T cells or NK cells producing IFNγ ( h ) or TNFα ( i ) in s.c. (black bars) or i.p. (grey bars) tumours from WT mice was assessed by intracellular staining 4 h after Brefeldin A injection. n =3–5 per group. Data (mean+s.e.m.) are representative of at least two independent experiments. ns: P >0.05, * P <0.05, ** P <0.01, *** P <0.001 by unpaired t -test ( b , e – i ) or one-way analysis of variance with Dunnett’s post test ( a , c ). Full size image Cytokine production differs between tumour sites Equivalent numbers of NK cells and CD8 T cells were present in both i.p. and s.c. tumours, demonstrating that NK induction of LN-like vasculature in s.c. but not i.p. tumours was not due to differential representation ( Fig. 5g ). To assess the effector activities of these cells, we treated tumour-bearing mice with Brefeldin A for 4 h and analysed the in vivo cytokine profiles immediately after harvest. About 20% of CD8 T cells in both tumour locations produced interferon-γ (IFNγ) ( Fig. 5h ). However, although ∼ 30% of NK cells in s.c. tumours produced IFNγ, <5% of NK cells in i.p. tumours did so ( Fig. 5h ). In addition, significantly larger fractions of NK cells and CD8 T cells produced tumour necrosis factor-α (TNFα) in s.c. tumours than in i.p. tumours ( Fig. 5i ). Thus, NK and effector CD8 T-cell functional activities depend on the location of tumour growth and the involvement of NK cells in inducing LN-like vasculature correlates with their secretion of IFNγ. IFNγ controls CCL21 but not PNAd expression in i.p. tumours We therefore tested whether effector lymphocyte-derived IFNγ induced LN-like vasculature. Naive OT-I cells failed to infiltrate i.p. tumours in IFNγ −/− hosts or in WT mice treated with IFNγ-neutralizing antibody ( Fig. 6a,b ). However, infiltration into s.c. tumours in IFNγ −/− mice was unimpaired ( Fig. 6c ). Reconstitution of Rag2 −/− mice with IFNγ −/− CD8 T cells before tumour implantation failed to rescue infiltration of adoptively transferred naive OT-I into established i.p. tumours ( Fig. 6d ), even though the repleted IFNγ −/− CD8 T cells were present in tumours in normal numbers ( Fig. 6e ). Surprisingly, PNAd was still expressed on tumour vasculature in these mice ( Fig. 6f,g ). In contrast, Ccl21 expression was significantly reduced ( Fig. 6h,j ). Ccl19 expression was not significantly different in i.p. tumours from WT and IFNγ −/− mice ( Fig. 6i ), demonstrating that its low-level expression ( Fig. 1m ) was insufficient to mediate naive T-cell recruitment. Thus, IFNγ secretion by endogenous CD8 T effectors controls only one element of LN-like vasculature in i.p. tumours. 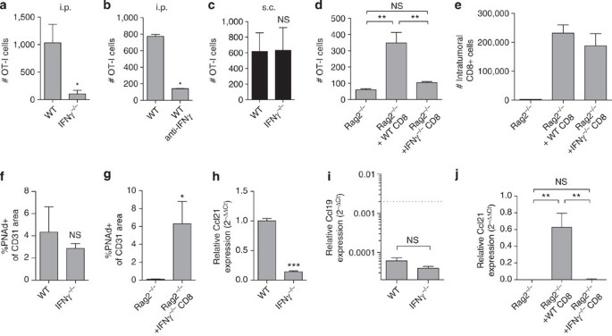Figure 6: IFNγ from endogenous CD8 T cells controls CCL21 but not PNAd expression in i.p. tumours. Infiltration of naive OT-I cells into i.p. (a,b,d) or s.c. (c) B16-OVA tumours in the indicated mice was determined as inFig. 2.n=7 (a), 3 (b,d) and 5 (c). Ind,Rag2−/−mice were repleted with either WT orIFNγ−/−CD8 T cells before tumour implantation. (e) The absolute number of CD8+T cells (non-OT-I) that had accumulated in i.p. B16-OVA tumours in mice with the indicated background was determined by flow cytometry.n=3 per group. (f,g) PNAd expression in i.p. tumours from the indicated mice was quantified as inFig. 3.n=3 per group.Ccl21(h,j) orCcl19(i) expression in i.p. tumours lysates from the indicated mice was quantified.Ccl21data (h,j) are presented as 2^−ΔΔCTmethod relative to HPRT with expression levels in control samples normalized to 1.Ccl19data (i) is presented as 2^−ΔCTrelative to HPRT. Dashed line representsCcl21expression levels in control tumours.n=3–6 per group. Data (mean+s.e.m.) are representative at least two independent experiments. ns:P>0.05, *P<0.05, **P<0.01, ***P<0.001 by unpairedt-test (a–c,f–i) or one-way analysis of variance with Tukey’s post test (d,j). Figure 6: IFNγ from endogenous CD8 T cells controls CCL21 but not PNAd expression in i.p. tumours. Infiltration of naive OT-I cells into i.p. ( a , b , d ) or s.c. ( c ) B16-OVA tumours in the indicated mice was determined as in Fig. 2 . n =7 ( a ), 3 ( b , d ) and 5 ( c ). In d , Rag2 −/− mice were repleted with either WT or IFNγ −/− CD8 T cells before tumour implantation. ( e ) The absolute number of CD8 + T cells (non-OT-I) that had accumulated in i.p. B16-OVA tumours in mice with the indicated background was determined by flow cytometry. n =3 per group. ( f , g ) PNAd expression in i.p. tumours from the indicated mice was quantified as in Fig. 3 . n =3 per group. Ccl21 ( h , j ) or Ccl19 ( i ) expression in i.p. tumours lysates from the indicated mice was quantified. Ccl21 data ( h , j ) are presented as 2^−ΔΔC T method relative to HPRT with expression levels in control samples normalized to 1. Ccl19 data ( i ) is presented as 2^−ΔC T relative to HPRT. Dashed line represents Ccl21 expression levels in control tumours. n =3–6 per group. Data (mean+s.e.m.) are representative at least two independent experiments. ns: P >0.05, * P <0.05, ** P <0.01, *** P <0.001 by unpaired t -test ( a – c , f – i ) or one-way analysis of variance with Tukey’s post test ( d , j ). Full size image IFNγ controls CCL21 expression by CD31 + and gp38 + cells In LN, CCL21 is produced by gp38 + CD31 neg fibroblastic reticular cells (FRCs), gp38 + CD31 + lymphatic endothelial cells (LECs) and gp38 neg CD31 + HEV [1] . Both i.p. and s.c. tumours contained gp38 + CD31 neg cells ( Fig. 7a ), which also expressed other markers of LN FRCs and fibroblasts, including CD140a, CD44 and VCAM-1 (ref. 38 ) ( Fig. 7b ). Tumours also contained CD31 + blood endothelial cells but very few gp38 + CD31 + LECs ( Fig. 7a ). Ccl21 was expressed by sorted gp38 + fibroblasts and CD31 + endothelial cells ( Fig. 7c ). All other examined cells, including CD45 neg gp38 neg CD31 neg cells (which includes tumour cells), CD11c + DCs and other CD45 + cells, expressed little to no Ccl21 ( Fig. 7c ). Based on cell numbers and per cell expression, gp38 + cells were the major source of CCL21 in both i.p. and s.c. tumours. Both gp38 + and CD31 + cells also expressed IFNγR1 ( Fig. 7d ), suggesting they could respond directly to IFNγ. Indeed, Ccl21 expression by both of these radioresistant cells was significantly decreased in i.p. tumours from WT→ IFNγR1 −/− bone marrow chimeras, compared with reciprocal chimeras in which only haematopoietic cells lacked IFNγR1 ( Fig. 7e ). These data support a model in which IFNγ secreted by CD8 effectors in i.p. tumours directly induces CCL21 in both gp38 + fibroblasts and endothelial cells. 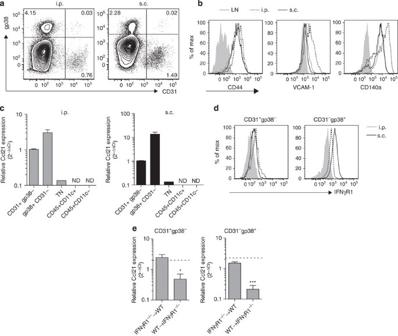Figure 7: IFNγ controls CCL21 expression by endothelial cells and gp38+cells. (a) Frequency of gp38+and CD31+cells among live singlet Ter119negCD45negcells from i.p. and s.c. tumours was determined by flow cytometry. (b) The phenotype of gp38+cells from LN (solid grey lines), s.c. (solid black lines) and i.p. (dotted lines) B16-OVA tumours was determined by flow cytometry by staining with the indicated markers. The parent gate is live singlet CD45neggp38+CD31neg. Shaded regions represent background staining in FMO controls. (c)Ccl21expression in the indicated purified cell populations from i.p. and s.c. tumours was measured by reverse transcriptase–PCR (RT–PCR). Expression levels in CD31+endothelial cells for each tumour location were normalized to 1. TN=CD45neggp38negCD31neg.n=3. nd=not detected. (d) IFNγR1 expression on CD31+and gp38+cells from i.p. (dashed lines) and s.c. (solid lines) tumours was determined by flow cytometry. Shaded regions represent background staining in FMO controls. (e)Ccl21expression in purified cell populations isolated from i.p. tumours inIFNγR1−/−→WTandWT→IFNγR1−/−bone marrow chimeras was measured by RT–PCR. Expression levels are presented relative toHprt. Dashed lines represent expression levels in WT→WT control chimera.n=4 per group. Data (mean+s.e.m.) are representative of three (a–d) independent experiments or one experiment (e). ns:P>0.05, *P<0.05, ***P<0.001 by unpairedt-test. Figure 7: IFNγ controls CCL21 expression by endothelial cells and gp38 + cells. ( a ) Frequency of gp38 + and CD31 + cells among live singlet Ter119 neg CD45 neg cells from i.p. and s.c. tumours was determined by flow cytometry. ( b ) The phenotype of gp38 + cells from LN (solid grey lines), s.c. (solid black lines) and i.p. (dotted lines) B16-OVA tumours was determined by flow cytometry by staining with the indicated markers. The parent gate is live singlet CD45 neg gp38 + CD31 neg . Shaded regions represent background staining in FMO controls. ( c ) Ccl21 expression in the indicated purified cell populations from i.p. and s.c. tumours was measured by reverse transcriptase–PCR (RT–PCR). Expression levels in CD31 + endothelial cells for each tumour location were normalized to 1. TN=CD45 neg gp38 neg CD31 neg . n =3. nd=not detected. ( d ) IFNγR1 expression on CD31 + and gp38 + cells from i.p. (dashed lines) and s.c. (solid lines) tumours was determined by flow cytometry. Shaded regions represent background staining in FMO controls. ( e ) Ccl21 expression in purified cell populations isolated from i.p. tumours in IFNγR1−/−→WT and WT→IFNγR1−/− bone marrow chimeras was measured by RT–PCR. Expression levels are presented relative to Hprt . Dashed lines represent expression levels in WT→WT control chimera. n =4 per group. Data (mean+s.e.m.) are representative of three ( a – d ) independent experiments or one experiment ( e ). ns: P >0.05, * P <0.05, *** P <0.001 by unpaired t -test. Full size image LTα 3 -TNFR signalling induces PNAd on tumour vasculature It remained unclear how effector lymphocytes induced PNAd expression on tumour vasculature independently of LTβR and IFNγ. Although TNFα was also secreted by endogenous effector lymphocytes ( Fig. 5 ), PNAd expression and naive T-cell infiltration were normal in i.p and s.c. tumours grown in TNFα −/− hosts ( Fig. 8a–c ). In contrast, PNAd expression and naive T-cell infiltration were significantly decreased in tumours growing in TNF receptor 1/2 ( TNFR1/2 −/− ) dual knockout hosts ( Fig. 8a–d ). Ccl21 levels were also significantly reduced ( Fig. 8e ). This suggested that homotrimeric LTα 3 , the other known ligand for TNFR1 and TNFR2, was responsible for inducing PNAd on tumour vasculature. Effector CD8 T cells sorted from i.p. and s.c. tumours expressed Lta mRNA at higher levels than Tnfa ( Fig. 8f ). We repleted Rag1 −/− mice with TNFα −/− or LTα −/− CD8 T cells and evaluated PNAd expression on subsequently implanted i.p. tumour vasculature. Representation of all repleted endogenous CD8 T cells in tumours was comparable to that of controls ( Fig. 8g ). TNFα −/− CD8 T cells restored PNAd to levels seen in tumours from WT mice ( Fig. 8h ). LTα −/− CD8 T cells, however, failed to significantly induce PNAd expression ( Fig. 8h ). Intratumoral CD31 + endothelial cells expressed TNFR1 but little TNFR2 ( Fig. 8i ). Using WT→ TNFR1/2 −/− and reciprocal bone marrow chimeras, PNAd expression on i.p. tumour vasculature was deficient only when endothelial cells did not express TNFRs ( Fig. 8j ). These results suggest a model in which LTα 3 released by effector lymphocytes directly engages TNFR1 on tumour endothelium to induce PNAd expression. 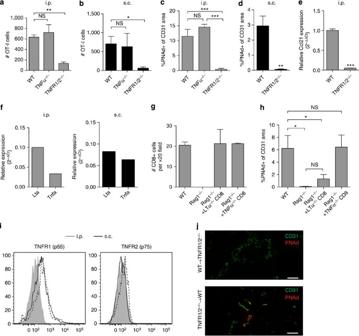Figure 8: LTα3induces PNAd expression on tumour vasculature by signalling through TNFRs. Infiltration of naive OT-I cells into i.p. (a) or s.c. (b) B16-OVA tumours in the indicated mice was determined.n=7 (a) or 4 (b) per group. PNAd expression (c,d) andCcl21expression in i.p. (c,e) or s.c. (d) tumours were quantified.n=4 per group. (f) Expression ofLtaandTnfamRNA in sorted CD3+CD8+T cells from i.p. (left panel) and s.c. (right panel) tumours was determined by quantitative reverse transcriptase–PCR. Expression levels are displayed relative toHprt. (g) Endogenous CD8 T-cell accumulation in day 14 i.p. B16-OVA tumours growing in WT,Rag1−/−andRag1−/−mice repleted with eitherTNFα−/−orLTα−/−CD8 T-cells (n=3 per group) was determined by immunofluorescence. (h) PNAd expression in i.p. tumours from the indicated mice was determined.n=4 per group. (i) Expression of TNFR1 and TNFR2 on CD31+endothelial cells from i.p. (dashed lines) and s.c. (solid lines) B16-OVA tumours was determined by flow cytometry. Shaded region represents background staining in FMO controls. (j) CD31 and PNAd expression in i.p. tumours fromWT→TNFR1/2−/−orTNFR1/2−/−→WTbone marrow chimeras. Data (mean+s.e.m.) are pooled from two experiments (a,b) or representative of two (c–j) independent experiments. ns:P>0.05, *P<0.05, **P<0.01, ***P<0.001 by unpairedt-test (d,e) or one-way analysis of variance with Tukey’s post test (a–c,h). Scale bars=100 μm. Figure 8: LTα 3 induces PNAd expression on tumour vasculature by signalling through TNFRs. Infiltration of naive OT-I cells into i.p. ( a ) or s.c. ( b ) B16-OVA tumours in the indicated mice was determined. n =7 ( a ) or 4 ( b ) per group. PNAd expression ( c , d ) and Ccl21 expression in i.p. ( c , e ) or s.c. ( d ) tumours were quantified. n =4 per group. ( f ) Expression of Lta and Tnfa mRNA in sorted CD3 + CD8 + T cells from i.p. (left panel) and s.c. (right panel) tumours was determined by quantitative reverse transcriptase–PCR. Expression levels are displayed relative to Hprt . ( g ) Endogenous CD8 T-cell accumulation in day 14 i.p. B16-OVA tumours growing in WT, Rag1 −/− and Rag1 −/− mice repleted with either TNFα −/− or LTα −/− CD8 T-cells ( n =3 per group) was determined by immunofluorescence. ( h ) PNAd expression in i.p. tumours from the indicated mice was determined. n =4 per group. ( i ) Expression of TNFR1 and TNFR2 on CD31 + endothelial cells from i.p. (dashed lines) and s.c. (solid lines) B16-OVA tumours was determined by flow cytometry. Shaded region represents background staining in FMO controls. ( j ) CD31 and PNAd expression in i.p. tumours from WT→TNFR1/2 −/− or TNFR1/2 −/− →WT bone marrow chimeras. Data (mean+s.e.m.) are pooled from two experiments ( a , b ) or representative of two ( c – j ) independent experiments. ns: P >0.05, * P <0.05, ** P <0.01, *** P <0.001 by unpaired t -test ( d , e ) or one-way analysis of variance with Tukey’s post test ( a – c , h ). Scale bars=100 μm. Full size image Tumour-infiltrating naive T cells delay tumour outgrowth We next determined whether naive T cells that infiltrated tumours via LN-like vasculature exerted a positive or negative effect after differentiating in the tumour mass. We transferred naive OT-I cells into C57BL/6 or TNFR1/2 −/− mice bearing early (day 8) s.c. B16-OVA tumours and monitored outgrowth and survival. At the time of naive T-cell transfer, we also initiated daily treatment with the sphingosine 1-phosphate receptor modulator FTY720, which efficiently prevents the egress of naive and activated lymphocytes from secondary lymphoid organs [39] , [40] , [41] , [42] . This setup allowed early infiltration of endogenous effectors necessary to induce LN-like vasculature, but prevented their ongoing egress from tumour draining LN into the tumour mass after the time of naive T-cell transfer. It also prevented the tumour infiltration of OT-I T cells that became activated in tumour draining LN. Thus, it allowed us to assess the activity of naive OT-I T cells that directly infiltrated the tumour via LN-like vasculature. The efficacy of FTY720 treatment was confirmed by examining the percentage of OT-I cells expressing high levels of CD44, a marker of antigen experience, in different LN beds. This percentage was high and similar in the tumour-draining inguinal LN of vehicle-treated and FTY720-treated mice ( Fig. 9a ). However, CD44-expressing OT-I cells in the antigen-free mesenteric LN, which redistribute from the tumour-draining LN [42] , were reduced by over 80% by FTY720 treatment ( Fig. 9a ). Despite sequestration of LN-activated effector T cells, naive OT-I cells that entered tumours in WT mice via LN-like vasculature significantly delayed tumour outgrowth and prolonged survival ( Fig. 9b,c ). In contrast, naive OT-I cells had no effect on tumours in TNFR1/2 −/− hosts, which lack LN-like vasculature ( Fig. 9b,d ). Thus, naive CD8 T cells that infiltrate tumours via LN-like vasculature enhance anti-tumour immunity. This is consistent with our previous demonstration that they become fully differentiated intratumoral effector cells [24] . 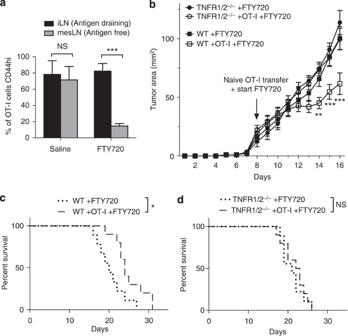Figure 9: Naive CD8 T cells that infiltrate tumours via LN-like vasculature delay tumour outgrowth. (a) WT mice with flank s.c. B16-OVA tumours received naive OT-I cells i.v. on day 8 after tumour implantation, and were given daily i.p. injections of either 1 mg kg−1FTY720 or saline beginning at the time of OT-I transfer. Draining inguinal LN (black bars) and non-draining mesenteric LN (grey bars) were harvested when tumours reached size limits. The percentage of OT-I cells expressing CD44 was determined by flow cytometry.n=5 per group. (b) WT orTNFR1/2−/−mice were implanted s.c. with B16-OVA tumors and received naïve OT-I cells or no T cells on day 8 after tumour implantation. All mice were treated daily with FTY720 beginning on day 8. Tumour size was monitored daily by caliper measurements, and tumour area (b) and survival (c,d) was determined.n=9 (no OT-I T cells) or 10 (OT-I T cells). Data (mean+s.e.m.) are representative of two independent experiments. ns:P>0.05, *P<0.05, **P<0.01, ***P<0.001 by unpairedt-test (a), two way analysis of variance (b) or log-rank test (c,d). Figure 9: Naive CD8 T cells that infiltrate tumours via LN-like vasculature delay tumour outgrowth. ( a ) WT mice with flank s.c. B16-OVA tumours received naive OT-I cells i.v. on day 8 after tumour implantation, and were given daily i.p. injections of either 1 mg kg −1 FTY720 or saline beginning at the time of OT-I transfer. Draining inguinal LN (black bars) and non-draining mesenteric LN (grey bars) were harvested when tumours reached size limits. The percentage of OT-I cells expressing CD44 was determined by flow cytometry. n =5 per group. ( b ) WT or TNFR1/2 −/− mice were implanted s.c. with B16-OVA tumors and received naïve OT-I cells or no T cells on day 8 after tumour implantation. All mice were treated daily with FTY720 beginning on day 8. Tumour size was monitored daily by caliper measurements, and tumour area ( b ) and survival ( c , d ) was determined. n =9 (no OT-I T cells) or 10 (OT-I T cells). Data (mean+s.e.m.) are representative of two independent experiments. ns: P >0.05, * P <0.05, ** P <0.01, *** P <0.001 by unpaired t -test ( a ), two way analysis of variance ( b ) or log-rank test ( c , d ). Full size image Organized lymphoid tissue develops in i.p. tumours As PNAd and CCL21 expression in inflamed tissues has been associated with formation of TLO, we determined whether this also occurred in tumours. In i.p. tumours, we found large follicular aggregates of B lymphocytes immediately surrounding some but not all sites of PNAd expression ( Fig. 10a ). These aggregates were co-extensive with a reticular network of gp38 + cells that did not stain for the LEC marker LYVE-1 ( Fig. 10a ), suggesting that they represented the gp38 + CD31 neg CCL21 + FRC-like cells identified by flow cytometry ( Fig. 7a ). T cells and DCs were also found in these structures, but they were not organized into a discreet zone ( Fig. 10b,c ), as has been seen in some TLO. Nonetheless, in conjunction with our earlier work [24] , these results suggest that organized lymphoid tissue associated with LN-like vasculature may serve as sites for the activation and regulation of recently entering naive T cells. 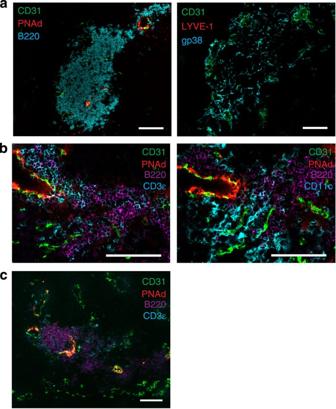Figure 10: LN-like vasculature is associated with organized lymphoid tissue in i.p. B16-OVA tumours. (a–c) i.p. B16-OVA tumours from C57BL/6 mice stained for the indicated cellular markers. Two adjacent sections were stained ina. Two different adjacent sections were stained inb. Images are representative of five tumours. Scale bars=100 μm. Figure 10: LN-like vasculature is associated with organized lymphoid tissue in i.p. B16-OVA tumours. ( a – c ) i.p. B16-OVA tumours from C57BL/6 mice stained for the indicated cellular markers. Two adjacent sections were stained in a . Two different adjacent sections were stained in b . Images are representative of five tumours. Scale bars=100 μm. Full size image Our observation of LN-like vasculature in multiple tumour models adds to a growing body of literature demonstrating its presence in mouse [21] , [23] and human [4] , [6] , [43] tumours. The presence of PNAd- and CCL21-positive LN-like vasculature in human tumours has been associated with a positive prognosis. We also previously showed that naive T cells enter tumours and differentiate into effectors [24] . Here we link these two observations, demonstrating that PNAd and CCL21 control naive T-cell entry into tumours. In contrast to LN HEV and many TLO models, development of intratumoral LN-like vasculature did not depend on LTβR signalling. Instead, it depended on other cytokines secreted by tumour-infiltrating CD8 or NK effector lymphocytes. PNAd on tumour endothelium was induced by LTα 3 signalling through TNFRs. CCL21 expression by endothelial cells and associated gp38 + fibroblasts was induced by IFNγ downstream of TNFR signalling in i.p. tumours. However, its control in s.c tumours is more complex. It probably involves IFNγ, which is made by both CD8 T cells and NK cells in these tumours and redundant factor(s) that remain to be identified. Interestingly, effector functions of intratumoral NK cells also varied with location of tumour growth, altering their ability to induce PNAd and CCL21 expression. Our results support a model in which an initial influx of LN-primed effector lymphocytes into the tumour induces the development of LN-like vasculature, which supports recruitment of naive T cells that contribute to ongoing anti-tumour immunity. Control of PNAd expression on LN HEV and in TLO models has been primarily attributed to DCs that express LTα 1 β 2 , which engages LTβR [7] , [8] , [13] , [14] . PNAd expression in human breast cancer has also been correlated with the presence of LTβ-producing DCs [22] . Other reports have also demonstrated a role for B cells in inflamed LN [44] , [45] and an indirect role for CD4 T cells by initiating DC-mediated induction of PNAd in a thyroiditis TLO model [18] . However, our results with mice deficient in effector lymphocyte populations clearly demonstrate that the simple presence of DCs is insufficient for inducing PNAd expression in B16 tumours. Similarly, neither B cells nor CD4 T cells are necessary or sufficient for inducing PNAd in this tumour model system. Instead, PNAd expression required endogenous effector CD8 T cells in i.p. tumours and either CD8 T cells or NK cells in s.c. tumours. Effector lymphocytes acted directly to induce PNAd by secreting LTα 3 , which engaged TNFRs on endothelial cells. The expression of TNFR1 rather than TNFR2 on endothelial cells in B16 tumours suggests that signalling through this receptor is responsible. Another recent report showed PNAd expression in methylcholanthrene-induced tumours required Treg depletion, although the molecular mechanism controlling PNAd expression was not defined [23] . However, in B16 tumours growing in WT mice and in genetically induced melanomas, PNAd is expressed despite the presence of Treg cells. Taken together, we suggest that the role of Tregs in regulating PNAd is indirect, by limiting the accumulation and/or effector activities, including LTα 3 secretion, of activated lymphocytes. The fact that Treg depletion was not required for PNAd expression in these melanoma models probably reflects in part the differences in antigenic strength between ovalbumin and neoantigens formed in genetically induced melanomas or methylcholanthrene-induced fibrosarcomas, tipping the balance towards more robust effector activity. Consistent with this, weakly antigenic B16-F1 tumours had reduced accumulation of effector lymphocytes and lower levels of PNAd expression than B16-OVA tumours. At the molecular level, LTβR signalling is critical for regulating PNAd expression on LN HEV [8] and in several TLO models [9] , [10] , [11] , [12] , [46] . Previous work by Ruddle and colleagues [15] , [16] , [47] , [48] also dissected the roles of LTα and LTβ, using a model of transgenic overexpression in the pancreas and kidney. In those studies, a primary role for LTβR signalling was also demonstrated, as PNAd + vasculature was not seen when the LTα transgene was expressed in the absence of LTβ [15] . Abluminal PNAd was present when only the LTα transgene was expressed in mice with endogenous LTβ, whereas luminal PNAd was dependent on transgenic expression of both LTα and LTβ [16] . In other circumstances, however, PNAd expression can be LTβR independent. For example, when LTβR is deleted from endothelial cells, PNAd remains present on cells that have otherwise lost the typical HEV morphology [49] . PNAd is also expressed on the abluminal surface of LN HEV in LTβ knockout animals [16] or mice treated with LTβR-Ig [8] , [45] . A role for LTα 3 -TNFR signalling in controlling this residual abluminal PNAd has been suggested [16] but not directly demonstrated. Here we have shown that PNAd expression on tumour-associated LN-like vasculature is LTβR independent and LTα 3 -TNFR dependent. Other characteristics of LN-like vasculature in tumours differ from LN HEV or other TLO models. First, PNAd expression levels on tumour vasculature are low compared with LN HEV, and PNAd in tumours was largely expressed on flat endothelium. Importantly, LTα 3 -induced PNAd on tumour vasculature was clearly luminal, enabling L-selectin-mediated naive T-cell infiltration that could be blocked by i.v. administration of PNAd antibody. LN-like vasculature co-expressed MAdCAM-1, which is found on HEV in mesenteric LN and is also induced by LTα 3 (refs 15 , 47 ). MAdCAM-1 did not contribute to naive T-cell infiltration, however, perhaps because it is not properly posttranslationally modified to serve as an L-selectin ligand. A critical step in the generation of PNAd is the sulfation of core glycoproteins by the sulfotransferases GlcNAc6ST-1 and GlcNAc6ST-2 (ref. 50 ). GlcNAc6ST-2 is expressed specifically in HEV and is primarily responsible for generating luminal PNAd [51] . GlcNAc6ST-1 is expressed more widely and contributes to both luminal and abluminal PNAd [52] , [53] , [54] . Our finding of low-level expression of PNAd on both luminal and abluminal surfaces suggest the induction of GlcNAc6ST-1 rather than GlcNAc6ST-2, by LTα 3 -TNFR signalling. In any case, molecular control of PNAd expression on tumour vasculature appears distinct from what has been reported in other systems, perhaps as a consequence of disregulated angiogenesis. A second component of LN HEV expressed on tumour vasculature was the chemokine CCL21. CCL21 expression has also been reported in human tumours [3] , [4] , [6] , but similar to PNAd its regulation and role in the tumour microenvironment is poorly understood. CCL21 expression depends on TNFα and LT in the spleen [55] , [56] and transgenic TLO models [16] , [57] , but its expression in adult LN is independent of these cytokines [8] , [45] , and no alternative regulatory mechanisms have been defined. In tumours CCL21 expression was controlled by effector lymphocytes, and in i.p. tumours both TNFR signalling and CD8 effector secretion of IFNγ were required. We are not aware of other reports that CCL21 is induced by IFNγ. In fact, one report demonstrated that IFNγ was required for a transient drop in CCL21 levels in the inflamed spleen [58] . Nevertheless, our data suggest that IFNγ directly induces CCL21 expression in both endothelial cells and gp38 + cells associated with LN-like vasculature. As i.p. tumours in TNFR1/2 −/− mice lack both PNAd and CCL21, while i.p. tumours in IFNγ −/− mice are deficient in CCL21 only, initial LTα 3 -TNFR signalling may enable subsequent responsiveness of CCL21 expression to IFNγ signalling. CCL21 expression by gp38 + cells is intriguing, because these cells share phenotypic characteristics with LN FRCs [38] , which are a major source of CCL21 in LN. gp38 + cells were also the major source of CCL21 in tumours, but were in proximity to PNAd + endothelial cells that also expressed CCL21 on their own. Thus, CCL21 displayed on LN-like vasculature that enables naive T-cell entry probably reflects both direct production by the endothelium and CCL21 transcytosed [59] from adjacent gp38 + cells. We also found that these gp38 + cells are organized around portions of LN-like vasculature into reticular networks in conjunction with large aggregates of B lymphocytes in i.p. tumours. The functionality of gp38 + cells as components or organizers of these TLO-like structures, the functionality of the structures themselves and the reasons they develop at only some sites of LN-like vasculature remain to be defined. Nonetheless, these observations point towards a level of immune organization within tumours that may offer additional targets for intervention. The cellular and molecular differences in induction of LN-like vasculature in i.p. and s.c. tumours highlight a microenvironmental heterogeneity that depends on the location of growth. This is typified by the greater secretion of IFNγ and TNFα by NK cells in s.c. tumours, enabling them to induce LN-like vasculature in this location. The enhanced functionality of NK cells in s.c. tumours could reflect the recruitment of distinct NK subpopulations that cannot reach i.p. tumours based on differential expression of chemokine receptors [60] . Alternatively, each location may display different levels of activating or inhibitory NK receptor ligands [61] , shifting the balance in s.c. tumours towards NK-cell activation. The presence of immunosuppressive cytokines in i.p. tumours such as TGFβ could also inhibit NK-cell effector activities. These differences may be driven by properties of the tumour microenvironment that are determined by external cues, as has been described in the regional control of DC programming of tissue selective T-cell trafficking [62] . Location-based microenvironmental heterogeneity may affect efforts to enhance immune responses in various metastatic sites. Evidence for both positive and negative effects of LN-like vasculature on anti-tumour immunity have been reported in murine models [20] , [21] . In several human studies, PNAd and CCL21 expression have been associated with a positive prognosis [3] , [4] , [5] , [6] . As our results demonstrate that the level of LN-like vasculature is correlated with the extent of accumulation by endogenous effector lymphocytes that induce it, this prognostic association could simply reflect that the presence of LN-like vasculature is a proxy for effector lymphocyte infiltration. However, here we have shown that the development of LN-like vasculature directly supports an ongoing anti-tumour response by enabling the infiltration of naive CD8 T cells, which can differentiate into effector cells in the tumour microenvironment. It is important to note that our demonstration of this effect occurred in an experimental setup that necessarily eliminated the normal constant traffic of LN-activated effectors as well as any ongoing traffic of naive T cells into the tumour. The overall impact of a more sustained influx of naive tumour-infiltrating CD8 T cells may therefore be even greater. Thus, induction of LN-like vasculature in tumours has the potential to be a key contributor to anti-tumour immunity by generating a self-sustaining infiltration of T cells into the tumour mass. Mice Female C57BL/6 mice (NCI); OT-I Rag1 −/− , Rag2 −/− and TNFα −/− mice (Taconic); Thy1.1 congenic, β 2 M −/− , IFNγ −/− , Rag1 −/− , μMT −/− , IFNγR1 −/− , LTα −/− and TNFR1/2 −/− mice (Jackson); and CD1d −/− mice (gift from Victor Laubach, University of Virginia) were bred and maintained under specific pathogen-free conditions. All gene knockout mice were on a C57BL/6 background. Animals were used at ∼ 8–12 weeks of age. All protocols were approved by the University of Virginia Institutional Animal Care and Use Committee. Tumour cells and injections B16-F1 melanoma cells, variants expressing cytoplasmic ovalbumin (B16-OVA) or a chimeric major histocompatibility complex molecule that presents tyrosinase (B16-AAD), and LLC-OVA (a gift from E. Podack, University of Miami) (4 × 10 5 cells) were injected i.p. or s.c. Tumors were allowed to establish for ∼ 14 days prior to naïve T-cell transfer or other analyses. Paraffin embedded melanomas from BRAF V600E PTEN −/− mice and BRAF V600E PTEN −/− with an activating mutation in β-catenin [27] , [34] were a kind gift from Dr Marcus Bosenberg (Yale). Treatments of tumour-bearing mice Anti-IFNγ [63] (250 μg) was injected i.p. every 7 days beginning 1 day before tumour implantation. LTβR-Ig fusion protein [25] (100 μg) was injected i.p. every 4 days, beginning 1 day before tumour implantation. NK cells were depleted by injection of 100 μg anti-NK1.1 (PK136, BioXcell) every 3 days beginning 3 day before tumour implantation. For repletion of Rag −/− mice, CD8 T cells purified from pooled LN and spleen by magnetic bead enrichment on an autoMACS Cell Separator (Miltenyi Biotec) (5 × 10 6 cells) were injected i.v. ∼ 3 days before tumour implantation. Adoptive transfer of naive T cells Naive OT-I T cells isolated from pooled LN and spleen of OT-I RAG1 −/− /Thy1.1 mice (4 × 10 6 cells) or polyclonal CD8 + T cells pooled from LN and spleen of C57BL/6 mice and depleted of CD44-expressing cells by magnetic beads (Miltenyi) were injected into the lateral tail vein of recipients. In blocking experiments, cells were incubated with 100 ng ml −1 pertussis toxin (Sigma) for 1 h at 37 °C, or 100 μg of rat IgG (Jackson Immunoresearch), anti-CD62L (Mel-14, ATCC), or anti-CD11a (M17/4, BioXcell) or 50 μg of anti-CCR7 (4B12, eBioscience) and washed before injection. Luminal PNAd or MAdCAM-1 were blocked by injection of 100 μg of anti-MAdCAM-1 (MECA-367, BioXcell), anti-PNAd (MECA-79, BioLegend), or isotype Rat IgG or IgM i.v. 1 h before T-cell transfer. In some experiments, cells were labelled with Cell Trace Violet (Invitrogen) before transfer. Tissues were harvested 1 or 18 h after naive T-cell transfer. Flow cytometry and cell sorting LN were homogenized before staining. Tumours were incubated with 0.5 mg ml −1 Collagenase A (Roche) and 60 U ml −1 DNase I (Sigma-Aldrich) for 30 min at 37 °C, homogenized and lymphocytes isolated on Lympholyte-M (Cedarlane). Single-cell suspensions were treated with anti-CD16/32 (2.4G2, BioXcell) to block Fc receptors, and then with one or more of the following fluorescently conjugated antibodies (0.25–2 μg ml −1 ): CD8α (53-6.7), Thy1.1 (HIS51), CD69 (H1.2F3), CD25 (PC61.5), CD44 (IM7), IFN-γ (XMG1.2), TNFα (MP6-XT22), CD3ɛ (145-2C11), CD45 (30-F11), CD45.1 (A20), CD45.2 (104), CD11c (N418), CD11b (M1/70), TNFR2 (TR75-54), gp38 (8.1.1), CD31 (390), IFNγR1 (2E2), CD140a (APA5), VCAM-1 (429), NK1.1 (PK136), CD49b (DX5), Ter119 (all from eBioscience), CD4 (GK1.5) (BD Biosciences), Thy1.2 (30-H12) and TNFR1 (55 R-286; BioLegend). Live/Dead Aqua (Invitrogen) or 4,6-diamidino-2-phenylindole (Sigma) were used to exclude dead cells from analysis. Samples were run on a FACSCanto II (BD) and analysed using FlowJo software (TreeStar). For sorting experiments, single-cell suspensions of tumours were pre-enriched using magnetic beads and then sorted to high purity on an Influx cell sorter (BD) directly into RNAProtect (Qiagen). Blood endothelial cells were gated as live singlet Ter119 − CD45 − gp38 − CD31 + . Gp38 + cells were gated as live singlet Ter119 − CD45 − gp38 + CD31 − . In-vivo effector function Tumour-bearing mice were injected i.p. with 250 μg of Brefeldin-A (Sigma-Aldrich). Four hours later, tumour-infiltrating lymphocytes were isolated as described above and stained for surface molecule expression, then stained for intracellular IFN-γ or TNF-α by using CytoFix/CytoPerm (BD Biosciences). Immunofluorescence microscopy Tissues were flash frozen in liquid nitrogen, embedded in optimum cutting temperature compound and cut into 6-μm sections. Sections were fixed with acetone/ethanol and blocked with PBS/5% BSA, anti-CD16/32, 3% H 2 O 2 , 0.1% NaN 3 and Avidin/Biotin Blocking Kit (Vector Laboratories). Paraffin-embedded melanomas from BRAF V600E PTEN −/− mice were deparaffinized, rehydrated and subjected to heat-induced antigen retrieval for 20 min at 95 °C in citrate buffer, pH 6.0, before blocking steps. Sections were stained with biotinylated or fluorescence-conjugated antibodies (5–20 μg ml −1 ) to CD31 (390), ICAM-1 (YN1/1.7.4), CD11c (N418), CD3ɛ (145-2C11), CD8α (53-6.7), B220 (RA3–6B2), LYVE-1 (ALY7), gp38 (8.1.1), MAdCAM-1 (MECA-367), VCAM-1 (429) (eBioscience), PNAd (MECA-79; BioLegend), CCL21 (R&D Systems) antibodies or appropriate isotype control antibodies followed by peroxidase or fluorescent Streptavidin conjugates (Jackson Immunoresearch). PNAd and CCL21 signals in frozen tumour sections were amplified with Tyramide Signal Amplification Plus kits (PerkinElmer). PNAd signals in paraffin-embedded sections were detected using DAB/Ni substrate (Vector) and slides were counterstained in Hematoxylin QS (Vector). For luminal PNAd staining, 100 μg of MECA-79 or Rat IgM was injected i.v. 30 min before tumour harvest. Slides were mounted in SlowFade Gold (Invitrogen) and images collected on a Microphot-FXA (Nikon) with Qcolor 5 CCD camera (Olympus) or AxioImager with Apotome (Zeiss). Image analysis Quantification of CD31 + and PNAd + areas was performed using ImageJ software (NIH) on original fluorescence images taken at identical exposures across samples. Consistent thresholds were applied to each image to identify CD31 + and PNAd + pixels. The percentage of CD31 + pixels of total imaged area and the percentage of PNAd + pixels within the region of interest of CD31 + area was calculated. Quantification of CD8 T-cell infiltration was performed by counting the number of cells present per 20 × field. Multiple sections per tumour and random fields per section were used for analysis. For image presentation, brightness and contrast were linearly adjusted and colour-merged images were generated using Photoshop CS6 software (Adobe). Reverse transcriptase–PCR RNA and a blend of oligo (dT) and random hexamer primers were used to generate complementary DNA (iScript cDNA Synthesis Kit, BioRad). Amplification was performed using iQ SYBR Green Supermix (BioRad) on a MyiQ qPCR Detection System (BioRad) with the following programme: 95 °C for 10 min; 40 cycles of 95 °C for 30 s, 60 °C for 1 min. Primers used were the following: Hprt forward 5′-AGGTTGCAAGCTTGCTGGT-3′ and reverse 5′-TGAAGTACTCATTATAGTCAAGGGCA-3′; Ccl21 forward 5′-CAAGGGCTGCAAGAGAACTG-3′ and reverse 5′-TGTGAGTTGGACCGTGAACC-3′; Ccl19 forward 5′-GCCTCAGATTATCTGCCAT-3′ and reverse 5′-ATCATTAGCACCCCCCAGAG-3′; Lta forward 5′-AAACCTGCTGCTCACCTTGT-3′ and reverse 5′-AGAGAAGCCATGTCGGAGAA-3′; Tnfa forward 5′-CCAAAGGGATGAGAAGTTCC-3′ and reverse 5′-CACTTGGTGGTTTGCTACGA-3′. Data are presented as 2^ −ΔΔC t or 2^ −ΔC t relative to Hprt as described in legends. Bone marrow chimeras Mice were irradiated (650 rad × 2) and reconstituted with a minimum of 2 × 10 6 bone marrow cells depleted of CD4 + and CD8 + T cells by magnetic beads (Miltenyi Biotec). Chimeras were maintained on Sulfatrim (sulfamethoxazole/trimethoprim) water for 3 weeks and were allowed to reconstitute for at least 8 weeks before use. Tumour control B16-OVA tumours were implanted s.c. into WT or TNFR1/2 −/− mice. On day 8 after implantation, mice were injected i.v. with 4 × 10 6 OT-I/Thy1.1 cells depleted of CD44-expressing cells by magnetic beads and treated daily with 1 mg kg −1 FTY720 (a gift from V. Brinkmann, Novartis Pharma AG, Basel, Switzerland) in sterile saline i.p., or treated with FTY720 without receiving naive T cells. Tumour size was monitored daily by caliper measurements and mice were killed when tumours reached 16 mm in any one dimension. Statistical analysis P- values were calculated for comparisons between two groups by unpaired t -tests and for comparisons between three or more groups by one-way analysis of variance with post tests, to correct for multiple comparisons as indicated in legends. P <0.05 was considered statistically significant. All graphs and statistics were calculated using Graph Pad Prism version 6.0. How to cite this article: Peske, J. D. et al. Effector lymphocyte-induced lymph node-like vasculature enables naive T-cell entry into tumours and enhanced anti-tumour immunity. Nat. Commun. 6:7114 doi: 10.1038/ncomms8114 (2015).